Cancer-associatedSF3B1mutations affect alternative splicing by promoting alternative branchpoint usage Hotspot mutations in the spliceosome gene SF3B1 are reported in ∼ 20% of uveal melanomas. SF3B1 is involved in 3′-splice site (3′ss) recognition during RNA splicing; however, the molecular mechanisms of its mutation have remained unclear. Here we show, using RNA-Seq analyses of uveal melanoma, that the SF3B1 R625/K666 mutation results in deregulated splicing at a subset of junctions, mostly by the use of alternative 3′ss. Modelling the differential junctions in SF3B1 WT and SF3B1 R625/K666 cell lines demonstrates that the deregulated splice pattern strictly depends on SF3B1 status and on the 3’ss-sequence context. SF3B1 WT knockdown or overexpression do not reproduce the SF3B1 R625/K666 splice pattern, qualifying SF3B1 R625/K666 as change-of-function mutants. Mutagenesis of predicted branchpoints reveals that the SF3B1 R625/K666 -promoted splice pattern is a direct result of alternative branchpoint usage. Altogether, this study provides a better understanding of the mechanisms underlying splicing alterations induced by mutant SF3B1 in cancer, and reveals a role for alternative branchpoints in disease. Discovery of recurrent missense mutations in splicing factors in cancers revealed the importance of the spliceosome pathway as a direct actor in carcinogenesis and questioned functional roles and molecular mechanisms of these mutations. SF3B1 ( Splicing Factor 3B Subunit 1A ) encodes for a core component of the U2 small nuclear ribonucleoprotein (snRNP) complex of the spliceosome and is involved in early stages of splicing. Alterations in SF3B1 were initially discovered in myelodysplastic syndromes (MDSs) and chronic lymphocytic leukemia (CLL), together with other mutations of splicing factors, such as U2AF1 , SRSF2 and ZRSR2 (refs 1 , 2 , 3 ). Importantly, these genes encode proteins that are all involved in 3′-splice site recognition during RNA splicing [4] . It has been shown that SF3B1 is mutated in a significant proportion ( ∼ 20%) of uveal melanoma (UM), a rare malignant entity deriving from melanocytes from the uveal tract [5] , [6] , [7] , and in other solid tumours at lesser frequencies [8] , [9] . RNA splicing is a fundamental process in eukaryotes, which is carried out by the splicing machinery (spliceosome) composed of five snRNPs and additional proteins [10] . Introns contain consensus sequences that define the 5′ donor splice site (5′ss), branchpoint (BP) and 3′ acceptor splice site (3′ss), which are initially recognized by the U1 snRNP, SF1 protein and U2AF, respectively. U2AF is a heterodimer composed of U2AF2 (also known as U2AF65) and U2AF1 (also known as U2AF35), which recognize the poly-pyrimidine tract and the well-conserved AG dinucleotide sequence of 3′ss, respectively. After binding to the 3′ss, U2AF facilitates replacement of SF1 by U2 snRNP at the BP. Interaction between U1 and U2 snRNPs then triggers transesterification joining the 5′-end of the intron to the BP, most generally an adenosine located in a loosely defined consensus ∼ 25 nucleotides upstream of the 3′ss. The 5′ss and 3′ss are then ligated together and the branched intron is discarded [10] . SF3B1 mediates U2 snRNP recruitment to the BP by interacting with the intronic RNA on both sides of the BP and with U2AF [11] . Structurally, the SF3B1 protein has an N-terminal hydrophilic region containing U2AF-binding motif and a C-terminal region, which consists of 22 non-identical HEAT (Huntingtin, Elongation factor 3, protein phosphatase 2A, Targets of rapamycin 1) repeats. Cancer-associated mutations in SF3B1 are missense mutations with three major hotspots targeting the fifth, sixth and seventh HEAT repeats at codon positions R625, K666 and K700, respectively. Interestingly, K700 mutations are by far the most frequent in haematopoietic malignancies, whereas R625 mutations are prevailing in UM. These alterations affect residues that are predicted to be spatially close to one another and therefore might have a similar functional impact [1] . Recently, RNA-sequencing (RNA-Seq) analysis of CLL, breast cancer and UM showed that a global splicing defect in SF3B1 -mutated tumours consists in usage of cryptic 3′ss (hereafter called AG′) located 10 to 30 bases upstream of normal 3′ss, yet the underlying mechanism has remained poorly understood. It has been proposed that AG′ is located at the end of a sterically protected region in a specific region downstream the BP. Yet, not every potentially located AG′ was used in an SF3B1 MUT context [12] . In the present study, RNA-Seq analysis of 74 primary UMs, mutated or not for SF3B1, confirmed the SF3B1 MUT -promoted pattern identified by DeBoever et al . [12] , demonstrating the robustness of the deregulated pattern. By constructing in cellulo models, we show that SF3B1 MUT is the direct cause of the deregulated splice pattern and could be qualified neither as gain-of-function (that is, hyperactivity) nor loss-of-function, but rather as change-of-function mutants. Our experiments provided evidence that (i) mutant SF3B1 preferentially recognizes alternative BPs upstream of the canonical sites and (ii) the alternative 3′ss used in a SF3B1 MUT context are less dependent on U2AF. We propose a model of the SF3B1 MUT dysfunctions that sheds new light on the mechanism of splicing dysregulation in cancer. In addition, our data reveal a currently under-appreciated role for recently described alternative branch points [13] in alternative splicing and disease. SF3B1 mutations promote upstream alternative acceptors Following initial finding of recurrent mutations of SF3B1 gene in UM [5] , we set up an independent consecutive series of UM to analyse the effect of SF3B1 hotspot mutations. This series included 74 T2–T4 tumours of different histologic types (21 epithelioid cell, 18 spindle cell and 35 mixed cases) treated by primary enucleation. Thirty-eight cases (51%) subsequently developed metastases and 40 patients (54%) died. 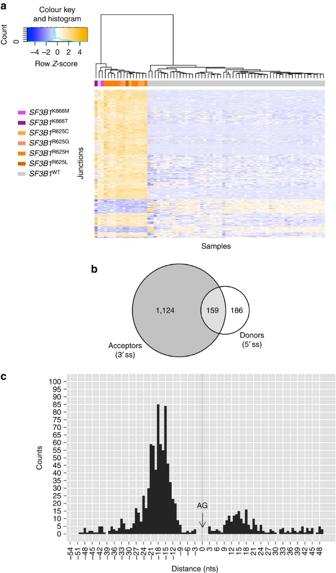Figure 1: Differential splice junctions inSF3B1MUTtumours. (a) Hierarchical clustering and heat-map analysis of differential splice junctions in tumour samples. The colours of squares below the tree denote the subtype of each sample. Below the array tree and the subtype identification row, the heat map of the 1,469 splice junctions is shown. The complete list of up- and downregulated splice junctions can be found inSupplementary Data 1. (b) Venn diagram of differential splice junctions inSF3B1MUTcompared withSF3B1WTtumours. Numbers show the count of alterations within only 5′ss (186 events) or only 3′ss (1,124 events). The overlapping area represents junctions that are either ambiguously attributed to an alternative donor or acceptor site, or attributed to both alternative 3′ and 5′ splice sites (159 events). (c) Distances between the alternative and canonicalSF3B1MUT-sensitive 3′ss. For alternative 3′ss within the 50 nts preceding the canonical 3′ss (765), the distance between the alternative (AG’) and corresponding canonical (AG) 3′ss was plotted as a histogram. Negative distances mean the alternative AG’ upstream of the canonical AG, whereas positive distances mean the AG’ downstream. The 0 point demarks the position of the canonical AG. SF3B1 mutations were found in 16 tumours affecting two hotspots p.R625 and p.K666 ( Supplementary Table 1 ). No mutation of other genes coding for splicing factors was observed. SNP array analysis did not reveal any chromosome loss or gain in the region containing SF3B1 (2q33.1). The overall mutation rate of 22% (16/74) is comparable to the rate (19%) recently reported for SF3B1 mutations in UM [5] , [6] , [7] . To evaluate the effects of SF3B1 mutations on splicing, we performed transcriptome analysis of the UM cohort using RNA-Seq technique. Differential analysis of splice junctions between the SF3B1 MUT ( n =16) and SF3B1 WT ( n =56) tumours using DESeq2 (ref. 14 ) revealed an overall high level of differences. The top 1,469 differentially spliced junctions with P -values ≤10 −5 (Benjamini-Hochberg) and absolute Log 2 (fold change)≥1 were selected for further analyses ( Supplementary Fig. 1 and Supplementary Data 1 ). A hierarchical clustering of the 74 tumours using the 1,469 differential splicing junctions showed coherent changes in SF3B1 MUT tumours ( Fig. 1a ). A single SF3B1 WT tumour clustered together with SF3B1 MUT cases. Manual reanalysis excluded any variant of its SF3B1- coding sequence or any over- or under-expression of the SF3B1 transcript and exome sequencing of this case failed to identify any mutation of the spliceosome genes as a potential genocopy. Figure 1: Differential splice junctions in SF3B1 MUT tumours. ( a ) Hierarchical clustering and heat-map analysis of differential splice junctions in tumour samples. The colours of squares below the tree denote the subtype of each sample. Below the array tree and the subtype identification row, the heat map of the 1,469 splice junctions is shown. The complete list of up- and downregulated splice junctions can be found in Supplementary Data 1 . ( b ) Venn diagram of differential splice junctions in SF3B1 MUT compared with SF3B1 WT tumours. Numbers show the count of alterations within only 5′ss (186 events) or only 3′ss (1,124 events). The overlapping area represents junctions that are either ambiguously attributed to an alternative donor or acceptor site, or attributed to both alternative 3′ and 5′ splice sites (159 events). ( c ) Distances between the alternative and canonical SF3B1 MUT -sensitive 3′ss. For alternative 3′ss within the 50 nts preceding the canonical 3′ss (765), the distance between the alternative (AG’) and corresponding canonical (AG) 3′ss was plotted as a histogram. Negative distances mean the alternative AG’ upstream of the canonical AG, whereas positive distances mean the AG’ downstream. The 0 point demarks the position of the canonical AG. Full size image Interestingly, 72% (1,060/1,469) of differential splice variants had no Ensembl Transcript identifiers (ENST) and these novel splice variants were found almost exclusively in SF3B1 mutants. To be noticed, only 9% (12,866/142,458) of non-differential splice variants had no ENST. The acceptor splice site (3′ss) was altered in 1,124 differential junctions (76.5%), whereas the altered donor splice site (5′ss) was observed in 186 differential junctions (12.7%; Fig. 1b ). For 159 junctions (10.8%), the novel junction was either ambiguously attributed to the alternative 5′ or 3′ss, or attributed to both alternative 5′ss and 3′ss. The analysis of distances between the alternative and canonical SF3B1 MUT -sensitive 3’ss showed repetitive peaks of alternative 3’ss every three nucleotides ( Fig. 1c ). Such spacing of two nucleotides suggests that frameshift variants are targeted by nonsense-mediated mRNA decay. We observed that the majority (765 out of 1,124) of the SF3B1 MUT -promoted alternative 3′ss—thereafter named AG′—were located within 50 nucleotides (nts) that precede the canonical 3′ss—thereafter named AG—with a clear clustering in the −12 to −24 nt region upstream of the canonical AG ( Fig. 1c ). No ENST Identifier exists for 675 out of these 765 AG′ alternative acceptor sites (88%). These results are concordant with a recent study based on RNA-Seq data from CLL, breast cancer and UM samples [12] . DeBoever et al . showed that 619 cryptic 3′ss clustering 10–30 nucleotides upstream of canonical 3′ss were used in cancers with SF3B1 mutations. Interestingly, we found 327 out of these 619 cryptic 3′ss (53%) to be differentially expressed in our data set, demonstrating the robustness of this splicing pattern despite the differences in the series of analysed tumours and bioinformatics pipelines. Sequence context determines acceptor sensitivity to SF3B1 MUT To validate the splice pattern detected in SF3B1 MUT tumours and to determine if it is conferred by sequences in the region of the 3′ss, we performed minigene splicing assay. We selected seven 3′ss within the top differential splice junctions associated with SF3B1 MUT tumours (named as sensitive 3′ss) and two 3′ss found unaltered in an SF3B1 MUT context (named as insensitive 3′ss; Table 1 ). Regions containing the selected 3′ss were cloned into an ExonTrap vector and expressed into human cell lines with different SF3B1 status: 2 UM cell lines, MP41 ( SF3B1 WT ) and Mel202 ( SF3B1 R625G ; Supplementary Figs 2 and 3 ). In addition, to directly determine whether the splice pattern detected in SF3B1 MUT tumours is dependent on SF3B1 status, we used two isogenic HEK293T cell lines, SF3B1 WT and SF3B1 K666T obtained by the CRISPR/Cas9 technology. RNA-Seq data, as visualized by IGV (Integrative Genomics Viewer), showed different mutation rates of 30% in Mel202 cells and 14% in SF3B1 K666T HEK293T cells, because of multiple copies of the wild-type SF3B1 allele in these aneuploid cell lines. As expected, Mel202 ( SF3B1 MUT ) clusters with the SF3B1 MUT tumours and MP41 ( SF3B1 WT ) clusters with SF3B1 WT tumours. Probably due to its low level of SF3B1 K666T expression, SF3B1 K666T -HEK293T clusters together with HEK293T (WT) and SF3B1 WT tumours ( Supplementary Fig. 2 ). Table 1 Sensitive and insensitive 3′ss selected for validation in cell lines. Full size table The splice forms corresponding to canonical AG usage were found expressed after transfection of the insensitive 3′ss constructs in all cell lines, regardless of their SF3B1 status ( Fig. 2a ). Likewise, for the seven sensitive 3′ss constructs, the splice forms corresponding to canonical AG usage were found expressed in the SF3B1 WT cell lines MP41 and HEK293T. By contrast, the SF3B1 MUT cell lines Mel202 and SF3B1 K666T HEK293T expressed the alternative splice forms using the alternative AG′ in addition to the canonical AG ( Fig. 2a ). The correspondence between band sizes and splice usage was verified by Sanger sequencing. Interestingly, the ratio of the alternative AG′ versus canonical AG usage (AG′/AG) based on capillary electrophoresis profiles varied according to the SF3B1 MUT /SF3B1 WT rate in the cell lines ( Fig. 2b,c ). Of note, a faint but significant usage of alternative AG′ in SF3B1 WT cell lines was detected on the capillary electrophoresis profiles for three sensitive 3′ss, ENOSF1 , TMEM14C and ZNF76 (AG′/AG in SF3B1 WT cell lines=0.2, 0.1 and 0.07, respectively), implying that the AG′ usage may be reinforced rather than induced de novo in an SF3B1 MUT context ( Fig. 2b ). 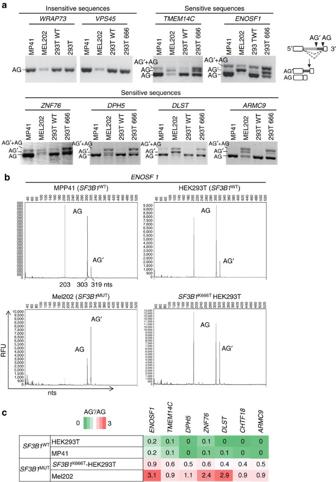Figure 2:In cellulovalidation of differential splice junctions. (a) Minigene splice assay of twoSF3B1MUT-insensitive 3′ss (WRAP73andVPS45) and 6SF3B1MUT-sensitive 3′ss (TMEM14C, ENOSF1, ZNF76, DPH5, DLST, ARMC9). Gel electrophoresis shows the different splicing processes for minigene ExonTrap constructions inSF3B1WTcell lines (MP41 and HEK293T) andSF3B1MUTcell lines (Mel202 and K666T-SF3B1HEK293T). The lower band corresponds to the variant generated by the usage of the canonical 3′ss (AG). The intermediate band corresponds to a splice generated by the usage of the alternative 3′ss (AG’). The upper band is the heteroduplex formation from two bands (AG and AG’). (b) Analysis of alternative AG’ and canonical AG usage of the ExonTrap construct (ENOSF1) in cell lines by capillary electrophoresis of RT–PCR products. Representative GeneMarker electrophoregrams for fragment analysis ofENOSF1minigene cDNA expression are shown. Thexaxis represents molecular size (in nucleotides (nts)) of PCR products, and theyaxis indicates relative fluorescent units (RFUs). The peak of 203 nts refers to the internal splicing of the pET01 ExonTrap vector using its 3′ss and 5′ss. The peak of 303 nts corresponds to the usage of the canonical AG, whereas the peak of 319 nts corresponds to the usage of alternative AG’ WT. (c) Heat-map analysis using the AG’/AG ratio of the top differential splice junctions in cell lines as determined by capillary electrophoresis of RT–PCR products. Figure 2: In cellulo validation of differential splice junctions. ( a ) Minigene splice assay of two SF3B1 MUT -insensitive 3′ss ( WRAP73 and VPS45 ) and 6 SF3B1 MUT -sensitive 3′ss ( TMEM14C, ENOSF1, ZNF76, DPH5, DLST, ARMC9 ). Gel electrophoresis shows the different splicing processes for minigene ExonTrap constructions in SF3B1 WT cell lines (MP41 and HEK293T) and SF3B1 MUT cell lines (Mel202 and K666T- SF3B1 HEK293T). The lower band corresponds to the variant generated by the usage of the canonical 3′ss (AG). The intermediate band corresponds to a splice generated by the usage of the alternative 3′ss (AG’). The upper band is the heteroduplex formation from two bands (AG and AG’). ( b ) Analysis of alternative AG’ and canonical AG usage of the ExonTrap construct ( ENOSF1 ) in cell lines by capillary electrophoresis of RT–PCR products. Representative GeneMarker electrophoregrams for fragment analysis of ENOSF1 minigene cDNA expression are shown. The x axis represents molecular size (in nucleotides (nts)) of PCR products, and the y axis indicates relative fluorescent units (RFUs). The peak of 203 nts refers to the internal splicing of the pET01 ExonTrap vector using its 3′ss and 5′ss. The peak of 303 nts corresponds to the usage of the canonical AG, whereas the peak of 319 nts corresponds to the usage of alternative AG’ WT. ( c ) Heat-map analysis using the AG’/AG ratio of the top differential splice junctions in cell lines as determined by capillary electrophoresis of RT–PCR products. Full size image In conclusion, we demonstrate that the aberrant splice pattern is strictly dependent on the SF3B1 MUT status and on sequences in the close vicinity of the sensitive 3′ss. SF3B1 hotspot mutations are change-of-function mutations The mode of action of SF3B1 mutant was then addressed by analysing endogenous DPH5 and ARMC9 transcripts. The different cell lines were transiently transfected with expression vectors for SF3B1 WT and SF3B1 K700E and examined 48 h later for the AG′/AG usage of endogenous 3′ss ( Fig. 3a ). We represent the shift from the canonical AG to the alternative AG′ by the AG′/AG index, which is the ratio of mRNA expression of AG′ form to AG form of a validated gene, DPH5 or ARMC9 , determined by quantitative reverse transcription (RT)–PCR. The overexpression of SF3B1 K700E significantly increased the AG′/AG index in SF3B1 WT cell lines (10- and 32-fold increases for DPH5 in MP41 and HEK293T, respectively), whereas overexpression of SF3B1 WT had no effect on the AG′/AG index. The overexpression of SF3B1 K700E increased by only three-fold the AG′/AG index in SF3B1 K666T HEK293T (transcript mutation rate=14%) and did not modify it in Mel202 cell line (transcript mutation rate=30%), which may indicate a saturating effect of SF3B1 MUT . Similar results were obtained with the endogenous sensitive 3′ss of ARMC9 . We conclude that SF3B1 mutation does not lead to a hyper-activity of the protein, as its phenotype is not reproduced by SF3B1 overexpression. 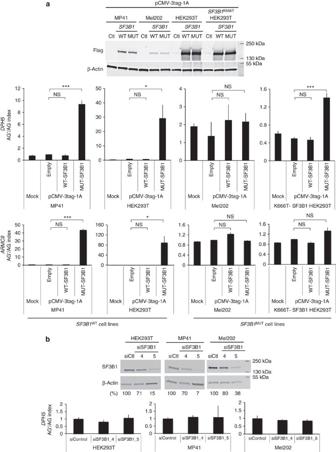Figure 3: Overexpression and underexpression of wild-typeSF3B1do not reproduce the splice pattern ofSF3B1hotspot mutations. (a) Effect of overexpression of wild-type and mutatedSF3B1on the AG’/AG ratio ofDPH5andARMC9inSF3B1WTandSF3B1MUTcell lines. MP41, Mel202, HEK293T andSF3B1K666T-HEK293T cell lines were transiently transfected with expression vectors forSF3B1WTandSF3B1K700E. The protein overexpression was confirmed by immunoblotting with anti-Flag using β-actin as a loading control (upper panel). Ratios of expression levels of alternative AG’ and canonical AG forms (AG’/AG) ofDPH5andARMC9were determined by quantitative RT–PCR (lower panel). The results are average of three replicates and are represented as mean±s.d. Pairedt-test was used to generate theP-values comparing each condition to the empty vector transfection: NS, non-significant; *P>0.05; ***P<0.001. (b) Effect of siRNA-mediated knockdown ofSF3B1on the AG’/AG ratio in cell lines. HEK293T, MP41 and Mel202 cells were transiently transfected with non-target control siRNA or two different siSF3B1: ‘4’and ‘5’. Proteins and RNA were extracted at 48 h after transfection. siRNA-mediated knockdown was confirmed by immunoblotting with anti-SF3B1, using anti-β-actin as a loading control. Numbers represent the protein band intensity normalized to β-actin and expressed as a percentage of control samples (upper panel). Ratios of expression levels of alternative AG’ form to the expression level of canonical AG form (AG’/AG) ofDPH5were determined by quantitative RT–PCR (lower panel). The results are average of three replicates and are represented as mean±s.d. Figure 3: Overexpression and underexpression of wild-type SF3B1 do not reproduce the splice pattern of SF3B1 hotspot mutations. ( a ) Effect of overexpression of wild-type and mutated SF3B1 on the AG’/AG ratio of DPH5 and ARMC9 in SF3B1 WT and SF3B1 MUT cell lines. MP41, Mel202, HEK293T and SF3B1 K666T -HEK293T cell lines were transiently transfected with expression vectors for SF3B1 WT and SF3B1 K700E . The protein overexpression was confirmed by immunoblotting with anti-Flag using β-actin as a loading control (upper panel). Ratios of expression levels of alternative AG’ and canonical AG forms (AG’/AG) of DPH5 and ARMC9 were determined by quantitative RT–PCR (lower panel). The results are average of three replicates and are represented as mean±s.d. Paired t -test was used to generate the P -values comparing each condition to the empty vector transfection: NS, non-significant; * P >0.05; *** P <0.001. ( b ) Effect of siRNA-mediated knockdown of SF3B1 on the AG’/AG ratio in cell lines. HEK293T, MP41 and Mel202 cells were transiently transfected with non-target control siRNA or two different si SF3B1 : ‘4’and ‘5’. Proteins and RNA were extracted at 48 h after transfection. siRNA-mediated knockdown was confirmed by immunoblotting with anti-SF3B1, using anti-β-actin as a loading control. Numbers represent the protein band intensity normalized to β-actin and expressed as a percentage of control samples (upper panel). Ratios of expression levels of alternative AG’ form to the expression level of canonical AG form (AG’/AG) of DPH5 were determined by quantitative RT–PCR (lower panel). The results are average of three replicates and are represented as mean±s.d. Full size image To determine whether SF3B1 mutations are loss-of-function mutations, we then assessed the effect of SF3B1 short interfering RNA (siRNA)-mediated knockdown on alternative splicing in SF3B1 WT HEK293T and MP41 and in SF3B1 MUT Mel202. Non-target siRNA was used as a negative control and siRNA-mediated knockdown was confirmed by immunoblotting ( Fig. 3b ). As shown in Fig. 3b , SF3B1 siRNA-mediated knockdown did not have any significant effect on AG′/AG index despite up to 93% of SF3B1 protein level reduction. These findings demonstrate that the SF3B1 MUT splice pattern is not mimicked by SF3B1 knockdown. Altogether, our results provide the first evidence that SF3B1 mutants are neither gain- (hyperactive) nor loss-of-function mutants, and suggest change-of-function consequences. SF3B1 MUT -promoted AG′ are weakly dependent on U2AF As sensitivity to SF3B1 mutants was conferred by sequences in the close vicinity of 3′ss ( Fig. 2 ), we searched for a sequence pattern associated with sensitive 3′ss. We compared the sequences of alternative AG′, corresponding canonical AG, and insensitive 3′ss ( Fig. 4a ). Two obvious features were found associated with AG′ consensus sequence: the paucity of G nucleotide at +1 position, and the frequency of A nucleotides at −11 to −14. Only 20% of G was observed for the alternative AG′, compared with ∼ 50% of G for both canonical AG and insensitive 3′ss ( Fig. 4b ). The high proportion of AG-(C/T) in the alternative AG′ site (65% versus 23% in AG′ and AG, respectively) is best explained by the presence of the AG′ within the polypyrimidine tract of the corresponding canonical AG. AG-G is part of the recognition motif of U2AF1 (ref. 15 ). The low frequency of G nucleotide immediately following alternative AG′ sites suggests lesser dependence to U2AF1 compared with the canonical AG at the step of 3’ss recognition [16] , [17] , [18] . To test this hypothesis, MP41 and HEK293T cells were transiently transfected with si U2AF1 or si U2AF2 . Efficient knockdown was confirmed by immunoblotting. As shown in Fig. 4c , both U2AF1 and U2AF2 knockdowns increased the AG′/AG index of DPH5 and ARMC9 in SF3B1 WT cells, and had no significant effect in SF3B1 R625/K666 cells ( Fig. 4c ). These findings suggest that AG′ is less dependent on U2AF than the competing canonical AG. 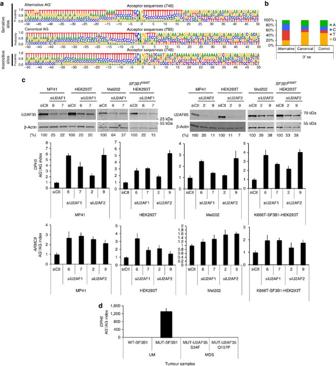Figure 4: Characterization of alternative 3′ss (AG’) sequences. (a) Comparison of sequence logos of 3′ss sensitive to SF3B1 status with canonical (AG) and alternative (AG’) sequences and 3′ss insensitive to SF3B1 status. One-hundred-nucleotide-long sequences surrounding the 3′ss were used to generate sequence logos with WebLogo. The height of each letter indicates the preference strength for that nucleotide at each position. (b) The proportion of the nucleotides immediately following the alternative (AG’), the canonical (AG) and insensitive 3′ss. (c) Effect ofU2AF35andU2AF65siRNA-mediated knockdown on the AG’/AG ratio in cell lines. MP41 and HEK293T (SF3B1WT) and Mel202 andSF3B1K666T-HEK293T (SF3B1MUT) cells were transiently transfected with non-target control siRNA, siU2AF35or siU2AF65. Proteins and RNA were extracted at 48 h after transfection. siRNA-mediated knockdown was confirmed by immunoblotting with anti-U2AF35 and anti-U2AF65, using anti-β-actin as a loading control. Numbers represent the protein band intensity normalized to β-actin and expressed as percentage of control samples (upper panel). Ratio of expression levels of alternative AG’ form to the expression level of canonical AG form (AG’/AG) ofDPH5andARMC9was determined by quantitative RT–PCR (lower panel). The results are average of three replicates and are represented as mean±s.d. (d) Effect ofU2AF35hotspot mutations on the AG’/AG ratio ofDPH5in MDS tumours. Ratio of expression levels of alternative AG’ form to the expression level of canonical AG form (AG′/AG) ofDPH5was determined by quantitative RT–PCR in two MDS samples, each harbouring one of the twoU2AF35hotspot mutations, S34F and Q157P and compared with mutated and wild-typeSF3B1uveal melanoma (UM) samples. Figure 4: Characterization of alternative 3′ss (AG’) sequences. ( a ) Comparison of sequence logos of 3′ss sensitive to SF3B1 status with canonical (AG) and alternative (AG’) sequences and 3′ss insensitive to SF3B1 status. One-hundred-nucleotide-long sequences surrounding the 3′ss were used to generate sequence logos with WebLogo. The height of each letter indicates the preference strength for that nucleotide at each position. ( b ) The proportion of the nucleotides immediately following the alternative (AG’), the canonical (AG) and insensitive 3′ss. ( c ) Effect of U2AF35 and U2AF65 siRNA-mediated knockdown on the AG’/AG ratio in cell lines. MP41 and HEK293T ( SF3B1 WT ) and Mel202 and SF3B1 K666T -HEK293T ( SF3B1 MUT ) cells were transiently transfected with non-target control siRNA, si U2AF35 or si U2AF65 . Proteins and RNA were extracted at 48 h after transfection. siRNA-mediated knockdown was confirmed by immunoblotting with anti-U2AF35 and anti-U2AF65, using anti-β-actin as a loading control. Numbers represent the protein band intensity normalized to β-actin and expressed as percentage of control samples (upper panel). Ratio of expression levels of alternative AG’ form to the expression level of canonical AG form (AG’/AG) of DPH5 and ARMC9 was determined by quantitative RT–PCR (lower panel). The results are average of three replicates and are represented as mean±s.d. ( d ) Effect of U2AF35 hotspot mutations on the AG’/AG ratio of DPH5 in MDS tumours. Ratio of expression levels of alternative AG’ form to the expression level of canonical AG form (AG′/AG) of DPH5 was determined by quantitative RT–PCR in two MDS samples, each harbouring one of the two U2AF35 hotspot mutations, S34F and Q157P and compared with mutated and wild-type SF3B1 uveal melanoma (UM) samples. Full size image One hypothesis to explain why U2AF knockdown partially mimicked the effect of SF3B1 MUT was that the SF3B1–U2AF2 interaction [11] might be decreased in the case of mutant SF3B1. However, U2AF2 and U2AF1 antibodies immunoprecipitated equally SF3B1 WT and SF3B1 K700M , implying no detectable alteration in the SF3B1 MUT –U2AF interaction ( Supplementary Fig. 4 ). Considering that U2AF1 mutations are reported in ∼ 10% of patients with MDS and associated with partial functional impairment in regulated splicing [2] , [19] , we tested two MDS samples each harbouring one of the two U2AF1 hotspot mutations, S34F and Q157P. Neither of these MDS samples presented any increase of the AG′/AG index of DPH5 , demonstrating that U2AF1 and SF3B1 hotspot mutations do not lead to the same aberrant splicing phenotype ( Fig. 4d ). Overall, our results exclude a defective SF3B1 MUT –U2AF interaction and show that U2AF1 MUT and SF3B1 MUT can induce different splicing patterns. Importantly, the rarity of G at the position +1 after AG′ as well as the increase of AG′/AG transcript ratio when U2AF is depleted suggest that SF3B1 MUT -promoted 3′ss (AG′) is less dependent on U2AF as compared with downstream canonical 3′ss (AG). Alternative BP usage in an SF3B1 MUT context The second feature characterizing the AG′ consensus sequence is the presence of frequent adenosines at a distance of 11–14 nts preceding the AG′, which could represent alternative BPs ( Fig. 4a ). Exploring this hypothesis, we investigated whether SF3B1 MUT alters BP choice. We used the online tools SVM (Support Vector Machine algorithm)-BPfinder and the Human Splicing Finder to predict the BP of the 744 sensitive 3′ss. The predicted BP clustered together at ∼ 22 nts upstream the insensitive 3′ss. However, the predicted BP for the alternative and canonical 3′ss showed a bi-modal distribution centred at 5 and 15 nts upstream the AG′, and at 20 and 35 nts upstream AG ( Fig. 5a ). Using the experimentally determined BP data set recently reported by Mercer et al . [13] , we found 286 out of the 744 sensitive 3’ss with a determined BP in an SF3B1 WT context ( Fig. 5a ). Remarkably, we found that 37% (105/286) of the A of the BP coincided with the A of AG′. Most of the other BP were closely distributed upstream of AG′ at an average of 5 nts. This superimposition of BP and AG′ made unlikely the usage of the same BP for both the canonical AG and alternative AG′. We thus suspected the usage of alternative branchpoint (BP′), possibly corresponding to the second peak of predicted BP around 35 nts 5′ to the AG and ∼ 15 nts 5′ to the AG′ ( Fig. 5a ). 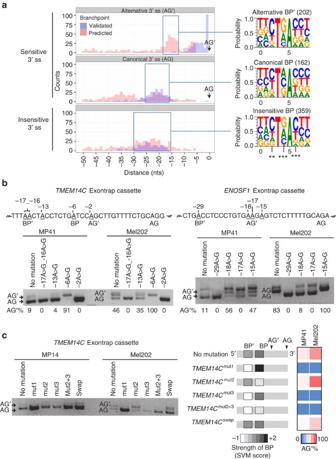Figure 5: Identification of alternative branchpoint usage in anSF3B1MUTcontext. (a) Analysis of distances between the branchpoints and the associated alternative (AG’), canonical (AG) or insensitive 3′ss. Left panel: Zero represents the position of the AG’, AG or insensitive 3′ss. Red bars represent the clusters of branchpoints predicted by the tool of SVM, blue bars represent the experimentally determined BP data set reported by Merceret al.13. Right panel: the extracted branchpoint sequence logos generated by WebLogo. **Significantly different in the three branchpoint patterns (χ2test,P<0.01), ***Significantly different in the three branchpoint patterns (χ2test,P<0.001). (b) Point mutations of branchpoints inTMEM14CandENOSF1ExonTrap constructs. All adenosines within a region of 30 nts preceding the canonical AG were mutated into guanines. Mutant constructs were expressed in MP41 (SF3B1WT) and Mel202(SF3B1MUT) cells followed by RT–qPCR. The lower band corresponds to the variant generated by the usage of the canonical 3′ss (AG). The intermediate band corresponds to the variant generated by the usage of the alternative 3′ss (AG’). The upper band is the heteroduplex formation from two bands (AG and AG′). The numbers represent the ratio of AG’ usage as determined by capillary electrophoresis. (c) Base-pairing potential mutants ofTMEM14C. Mutant constructs (sequences shown inSupplementary Fig. 5) were expressed in MP41 (SF3B1WT) and Mel202 (SF3B1MUT) cells followed by RT–qPCR. The lower band corresponds to the variant generated by the usage of the canonical 3′ss (AG). The upper band corresponds to the variant generated by the usage of the alternative 3′ss (AG’). A schematic presentation of the strength of the resulting branchpoints as estimated by their SVM score is shown on the right panel. The ratio of AG’ usage as determined by capillary electrophoresis in MP41 and Mel202 cells is shown as a heat map. Figure 5: Identification of alternative branchpoint usage in an SF3B1 MUT context. ( a ) Analysis of distances between the branchpoints and the associated alternative (AG’), canonical (AG) or insensitive 3′ss. Left panel: Zero represents the position of the AG’, AG or insensitive 3′ss. Red bars represent the clusters of branchpoints predicted by the tool of SVM, blue bars represent the experimentally determined BP data set reported by Mercer et al . [13] . Right panel: the extracted branchpoint sequence logos generated by WebLogo. **Significantly different in the three branchpoint patterns ( χ 2 test, P <0.01), ***Significantly different in the three branchpoint patterns ( χ 2 test, P <0.001). ( b ) Point mutations of branchpoints in TMEM14C and ENOSF1 ExonTrap constructs. All adenosines within a region of 30 nts preceding the canonical AG were mutated into guanines. Mutant constructs were expressed in MP41 ( SF3B1 WT ) and Mel202 (SF3B1 MUT ) cells followed by RT–qPCR. The lower band corresponds to the variant generated by the usage of the canonical 3′ss (AG). The intermediate band corresponds to the variant generated by the usage of the alternative 3′ss (AG’). The upper band is the heteroduplex formation from two bands (AG and AG′). The numbers represent the ratio of AG’ usage as determined by capillary electrophoresis. ( c ) Base-pairing potential mutants of TMEM14C . Mutant constructs (sequences shown in Supplementary Fig. 5 ) were expressed in MP41 ( SF3B1 WT ) and Mel202 ( SF3B1 MUT ) cells followed by RT–qPCR. The lower band corresponds to the variant generated by the usage of the canonical 3′ss (AG). The upper band corresponds to the variant generated by the usage of the alternative 3′ss (AG’). A schematic presentation of the strength of the resulting branchpoints as estimated by their SVM score is shown on the right panel. The ratio of AG’ usage as determined by capillary electrophoresis in MP41 and Mel202 cells is shown as a heat map. Full size image To explore such hypothesis, we mutated all adenosines within a region of 30 nts preceding the canonical AG in two sensitive sequences, TMEM14C and ENOSF1 . These two minigenes were selected for their low frequency of adenosines upstream the 3′ss in order to limit the number of required site-directed mutations. We then expressed these variant acceptor sequences in MP41 ( SF3B1 WT ) and Mel202 (SF3B1 MUT ) cells followed by RT–quantitative PCR and fragment analysis by capillary electrophoresis as described above ( Fig. 5b ). The observed consequences of TMEM14C mutants were the following: (i) the -17A>G_-16A>G-double mutation completely abolished the usage of the alternative AG′ in both recipient cell lines; (ii) the -13A>G mutation had no consequence on 3′ss usage; (iii) the -6A>G mutation completely abolished the usage of the canonical AG; (iv) the -2A>G mutation completely abolished the usage of the alternative AG′ as it destroyed the AG′ site. We interpret these data as indicating that the A at 30 nts upstream of AG is the BP′ for AG′, as its mutation allowed only the use of the canonical AG regardless of SF3B1 status. Alternatively, -6A>G mutation switched the usage of the AG to the usage of AG′, arguing that this site may serve as the BP for the canonical AG. Our data therefore support the existence of two branchpoints, BP and BP′, differentially used depending on the SF3B1 status. Similar observations were obtained with the ENOSF1 construct confirming the existence of two different BPs. Specifically, we could determine the BP′ of AG′ at 29 nts preceding the AG (-29A>G). The -18A>G mutation disturbed the usage of both AG′ and AG, whereas the -17A>G mutation disturbed AG usage and inhibited the usage of AG′. In fact, the later mutation created another alternative acceptor site replacing the AG′ (AAG>AGG), and competing with the canonical AG. The potential BP was loosely defined for ENOSF1 , because of the multiple adenosines in the vicinity of AG′ participating to the usage of the canonical AG. To be noticed, the -15A>G mutation of the nucleotide immediately following the AG′ strengthened the alternative site, presumably by reinforcing the binding of U2AF1 to the AG′-G site. Thus, the analyses of both the TMEM14C and ENOSF1 genes indicate that SF3B1 MUT affects the 3′ss choice by promoting the use of alternative BPs. SF3B1 plays a major role in U2 snRNP recruitment to the BP. To determine whether the potential of BP sequences to form base-pairing interaction with U2 snRNA (small nuclear RNAs) can modulate the sensitivity to SF3B1 mutations, BP and BP′ mutants of TMEM14C were generated ( Supplementary Fig. 5 ). The strength of the resulting BPs was estimated by their SVM score [20] ( Fig. 5c ). The TMEM14C mut1 allows a perfect base-pairing of BP with U2 snRNA [21] ; TMEM14C mut2 contains a suboptimal BP; TMEM14C mut3 contains a defective alternative BP′; TMEM14C mut2+3 includes both TMEM14C mut2 and TMEM14C mut3 mutated regions and TMEM14C swap contains swapped endogenous BP and BP′ sequences. The consequences of these mutants were then assessed by the AG′/AG index (RT–PCR). Enhancing the base-pairing of the BP region ( TMEM14C mut1 ), disrupting BP′ ( TMEM14C mut3 ) or combining a disrupted BP′ with a suboptimal BP ( TMEM14C mut2+3 ) led to a total inhibition of AG′ usage, regardless of the SF3B1 status. Decreasing the strength of BP ( TMEM14C mut2 ) led to a reinforcement of AG′ usage ( Fig. 5c ). Interestingly, swapping the BP and BP′ sequences ( TMEM14C swap ) decreased AG′ usage, which could be interpreted as a higher strength of BP′ as compared with BP to form base-pairing interactions with U2 snRNA. We extended this finding by an in silico comparison of the sequence patterns of alternative, canonical and insensitive BPs. We show that the canonical, alternative and insensitive BP presented distinct patterns ( Fig. 5a ), with significant sequence differences at positions +2, +4 and +6 of the motif (+5 being the A of the BP). These data suggest that SF3B1 MUT favours the use of BP′ with stronger base-pairing potential with U2 snRNA compared with the downstream BP. Collectively, in an SF3B1 MUT context, the stronger affinity of BP′ for U2 snRNA when compared with BP may allow the use BP′ with suboptimal AG′ (not followed by G, Fig. 4b ) and may explain the lower dependence of AG′ on U2AF ( Fig. 4c ). Here, we addressed the consequences of SF3B1 hotspot mutations on splicing in UM and its underlying mechanisms. First, we observed that SF3B1 hotspot mutations in UM are associated with deregulation of a restricted subset ( ∼ 0.5%) of splice junctions, mostly caused by the usage of alternative 3′ss (AG′) upstream of the canonical 3′ss (AG). This finding is concordant with a recent publication [12] , implying the robustness of the deregulated splice pattern in SF3B1 MUT tumours. Furthermore, this pattern is shared by tumours having for origin different cell lineages [12] , [22] . Second, we show here that SF3B1 MUT pattern was reproduced neither by knockdown nor by overexpressing wild-type SF3B1, indicating that SF3B1 mutants could be qualified as change-of-function mutants. Third, and important, our data provide significant progress in understanding the molecular mechanisms underlying alternative 3′ss regulation by SF3B1 MUT . We show that this mechanism involves a misregulation of BP′ usage, which have been largely overlooked in previous studies of alternative splicing and have been identified only recently on a large scale [13] . Based on in silico data, DeBoever et al . proposed that SF3B1 MUT -induced alternative 3′ss (AG′) is located at the end of a sterically protected region in a specific region downstream the canonical BP. Yet, not every potentially well-located AG′ was used in an SF3B1 MUT context, suggesting additional or different requirements for SF3B1 MUT selectivity [12] . They hypothesized no alternative BP usage as a mechanism of AG′ selection, because of the observed limited distances between AG and AG′. Strikingly, however, we showed here that mutagenesis of the predicted BP′ and the predicted canonical BP abrogated usage of AG′ and AG, respectively, confirming the existence of two BPs differentially used according to SF3B1 status. Interestingly, since submission of our work, Darman et al . reported findings fully confirming our results. They also showed the consequences of SF3B1 mutations on transcription through the generation of nonsense-mediated mRNA decay-sensitive aberrant spliced transcripts [23] . Until recently, only few examples of alternative branchpoints were reported, such as in human XPC and rat fibronectin genes [24] , [25] . However in 2015, the genome-wide identification of BPs revealed that one-third (32%) of introns have at least two BPs [13] , but little is known about their regulation. Our findings provide the first evidence that misregulation of alternative BPs is involved in physiology or pathology. Our findings indicate that SF3B1 MUT -induced alternative 3′ss usage relies on three properties: an AG′ with lower affinity to U2AF than the canonical 3′ss, the presence of an BP′ with a higher affinity to U2 snRNA than canonical BP and the location of BP′ at a distance of 11–14 nts preceding the AG′. Based on these findings and on current understanding of SF3B1 function, we propose the following model for how SF3B1 MUT exerts its effects ( Fig. 6 ). Because BP′ potential to form base-pairing interactions with U2 snRNA is generally superior to that of canonical BP, we suggest that U2 snRNP containing SF3B1 MUT has more stringent requirement for BP sequences than U2 snRNP-containing SF3B1 WT . Consistently, the hotspot mutations of SF3B1 target the HEAT repeats of SF3B1, which form helical structures that occlude the binding surface for RNA recognition motif of p14, a component of U2 snRNP that binds the BP [1] , [26] . The hotspot mutations of SF3B1 in the HEAT repeats occur on the inner surface of the structure and may induce a conformational change in the U2 snRNP complex altering its selectivity for BPs. It is likely that stronger BP′ (in terms of U2 snRNA complementarity) can compensate for lower AG affinity to U2AF, leading to the recognition of BP′ in a U2AF-independent manner (or less dependent than in the case of canonical BP). This model is supported by our U2AF depletion experiments and is consistent with previous findings that BP recognition may depend or not on AG binding to U2AF35, according to BP and 3′ss sequence and organization [11] , [16] , [17] , [18] . In contrast, SF3B1 WT may allow a more promiscuous binding of U2 snRNA to both canonical and alternative BPs, and in this case, the final choice of BP may be determined by context, especially 3′ss affinity for U2AF. 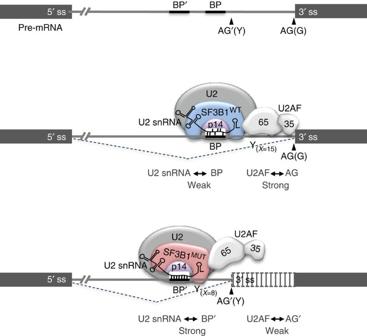Figure 6: A model for alternative splicing dysregulation induced bySF3B1hotspot mutations. The 3′ss contains a segment, which is rich in pyrimidines (Y), a well-conserved AG dinucleotide and a branchpoint (BP) sequence recognized by the U2 snRNP. The U2 snRNP complex binds to the intron through base-pairing interactions between the BP sequence and the U2 snRNA, and through interactions between intron sequences, SF3B1 and p14. The HEAT repeats of SF3B1 form helical structures that occlude the surface of RNA recognition motif of p14. U2 snRNP containing SF3B1WTrecognizes the canonical U2AF-dependant BP. The hotspot mutations ofSF3B1targeting the HEAT repeats occur on the inner surface of the structure and might induce a conformational change in the U2 snRNP complex altering its selectivity for BPs. U2 snRNP containing SF3B1MUThas more stringent requirement for BP sequences and less for U2AF-dependent sequences, leading to the binding of alternative branchpoints (BP’) with high potential of base-pairing with U2 snRNP. AG, canonical 3′ss; AG’, alternative 3′ss;x, average number of pyrimidines; Y, pyrimidine. Figure 6: A model for alternative splicing dysregulation induced by SF3B1 hotspot mutations. The 3′ss contains a segment, which is rich in pyrimidines (Y), a well-conserved AG dinucleotide and a branchpoint (BP) sequence recognized by the U2 snRNP. The U2 snRNP complex binds to the intron through base-pairing interactions between the BP sequence and the U2 snRNA, and through interactions between intron sequences, SF3B1 and p14. The HEAT repeats of SF3B1 form helical structures that occlude the surface of RNA recognition motif of p14. U2 snRNP containing SF3B1 WT recognizes the canonical U2AF-dependant BP. The hotspot mutations of SF3B1 targeting the HEAT repeats occur on the inner surface of the structure and might induce a conformational change in the U2 snRNP complex altering its selectivity for BPs. U2 snRNP containing SF3B1 MUT has more stringent requirement for BP sequences and less for U2AF-dependent sequences, leading to the binding of alternative branchpoints (BP’) with high potential of base-pairing with U2 snRNP. AG, canonical 3′ss; AG’, alternative 3′ss; x , average number of pyrimidines; Y, pyrimidine. Full size image Further work is required to evaluate the molecular mechanism by which the mutations of the SF3B1 HEAT domains may influence the base-pairing potential of U2 snRNA. The functional impact of SF3B1 MUT -deregulated splicing pattern on oncogenesis also remains to be understood. Meanwhile, our study opens new possibilities for applying the deregulated splicing pattern as a screening tool as well as for targeting the splicing deregulation as a therapeutic strategy in UM and other SF3B1 MUT -associated diseases [27] . Patient cohort A series of 109 consecutive patients diagnosed for UM without metastasis at diagnosis and treated by primary enucleation at the Institut Curie between January 2006 and December 2008 was assembled. RNA extracted from the tumour specimens was qualified for 74 (74/109) cases, which defined the patient cohort for this study. RNA samples were obtained from surgical residual tumour tissues. In accordance to the national law on the protection of individuals taking part in biomedical research, patients were informed by their referring oncologist that their biological samples could be used for research purposes and they gave their verbal informed consent. All analyses done in this work were approved by the Institutional Review Board and Ethics Committee of the Institut Curie Hospital Group. DNA and RNA sequencing Tumour DNA and RNA were provided by the Biological Resource Center of the Institut Curie. The DNA was extracted from frozen tumour or formalin-fixed paraffin-embedded samples using a standard phenol/chloroform procedure. SF3B1 was sequenced by Sanger methods as previously described [5] . Primers used for Sanger sequencing are: (forward) 5′-CCAACTCATGACTGTCCTTTCT-3′ and 5′-TGGAAGGCCGAGAGATCATT-3′. The total RNA was isolated from frozen tumour samples using a NucleoSpin Kit (Macherey-Nagel). cDNA synthesis was conducted with MuLV Reverse Transcriptase in accordance with the manufacturers’ instructions (Invitrogen), with quality assessments conducted on an Agilent 2100 Bioanalyzer. Libraries were constructed using the TruSeq Stranded mRNA Sample Preparation Kit (Illumina) and sequenced on an Illumina HiSeq 2500 platform using a 100-bp paired-end sequencing strategy. An average depth of global sequence coverage of 114 million and a median coverage of 112 million was attained. RNA-Seq analysis TopHat (v2.0.6) [28] was used to align the reads against the human reference genome Hg19 RefSeq (RNA sequences, GRCh37) downloaded from the UCSC Genome Browser ( http://genome.ucsc.edu ). Read counts for splicing junctions from junctions.bed TopHat output were considered. Differential analysis was performed on junction read counts using DESeq2 (ref. 14 ). Only alternative acceptor splice sites (two or more 3′ss with junctions to the same 5′ss) and alternative donor splice sites (two or more 5′ss with junctions to the same 3′ss) were considered for this analysis. Fifty-nucleotide-long sequences surrounding the splice acceptor sites were extracted to generate sequence logos using WebLog 3 ( http://weblogo.threeplusone.com/ ) [29] with the default parameters, the classic colour scheme and the unit frequency being plotted as ‘probability’. The data set supporting the results of this article is available on ArrayExpress repository under the accession E-MTAB-4097. BP sequence analysis The online tools SVM-BPfinder [20] ( http://regulatorygenomics.upf.edu/Software/SVM_BP/ ) and the Human Splicing Finder [30] ( http://www.umd.be/HSF/ ) were used to predict the BPs. The SVM_BP code was altered to allow for BP six base pairs from the 3′ss by setting minidist3ss=6 in svm_getfeat.py. Minigene constructs For each selected candidate gene alternative AG′-centred sequence of ∼ 200 nucleotides was PCR amplified from the genomic DNA of HEK293T cells using Phusion Hot Start II High Fidelity DNA Polymerase (Thermo Fisher Scientific). The primer sequence information is provided in Supplementary Table 2 . We introduced 15 bases of homology with the ends of the linearized vector at the 5′-end of the forward and reverse primers. Using In-fusion HD cloning kit (Clontech), we cloned the amplicon into the Bam H1 site of pET01 ExonTrap vector (Mobitec) containing a functional splice donor site ( Supplementary Fig. 3 ). Wild-type and mutated SF3B1 constructs A pCMV-3tag-1A vector containing wild-type SF3B1 was synthesized by Genscript Corporation. Because mammalian SF3B1 cDNA sequence was found unclonable in bacteria, a synthetic sequence was generated after codon-optimization for expression in bacteria. The full sequence of codon-optimized SF3B1 is available upon request. K700E mutation in SF3B1 was introduced using QuikChange II Site Directed Mutagenesis Kit (Stratagene). All constructs were verified by DNA sequencing. Primers used for generating the mutated SF3B1 are: (forward) 5′-CTGGTGGATGAGCAGCAGGAGGTCAGAACCATCTCTGC-3′ and (reverse) 5′-GCAGAGATGGTTCTGACCTCCTGCTGCTCATCCACCAG-3′. BP mutant constructs Mutations of potential BP in TMEM14C and ENOSF1 ExonTrap constructs were introduced using QuikChange II Site Directed Mutagenesis Kit (Stratagene) and verified by DNA sequencing. The primer sequences used to generate the mutations are provided in Supplementary Table 3 . Cell culture and transfection Mel202 cell line was purchased from the European Searchable Tumour Line Database (Tubingen University, Germany) and MP41 (derived at Institut Curie and described in ref. 31 ) UM cell lines were cultured in RPMI-1640 supplemented with 10% fetal bovine serum. A point mutation in SF3B1 resulting in K666T amino-acid substitution was introduced using CRISPR/CAS9-stimulated homology-mediated repair to generate isogenic HEK293T cell lines and was verified by Sanger sequencing. A donor template encoding a puromycin selection cassette was transfected at a 1:1:1 ratio with Cas9 (Addgene 41815) and a SF3B1 -specific gRNA (built from gRNA cloning vector, Addgene 41824). The selection cassette was removed by flippase-mediated excision. All cell lines were tested and proved to be Mycoplasma free. Authentication of the cell lines was verified by Sanger sequencing for their mutational status and by RNA-Seq. Plasmid transfections were carried out in cell lines using 500 ng of plasmid construct and LipofectAMINE 2000 reagent (Invitrogen) according to the manufacturer’s instructions. After 24 h, total RNA was extracted with NucleoSpin RNA kit (Macherey-Nagel). The quantity and quality of RNA was determined by spectrophotometry (NanoDrop Technologies). Five hundred nanograms of RNA was used as a template for cDNA synthesis with the High Capacity cDNA Reverse Transcription Kit (Applied Biosystems). Twenty-five nanograms of the synthesized cDNA was used as a template for RT–PCR amplification with specific primers. HEK293T and MP41 cells were transfected with the following siRNA obtained from Qiagen: SF3B1 (Cat.No. SI00715932 and Cat. No. SI04154647), U2AF1 (Cat.No. SI04158049 and Cat. No. SI04159547); U2AF2 (Cat.No. SI00754026 and Cat. No. SI04194498) or control siRNA (Cat.No. S103650318). The cells were transfected with 50 nM of siRNA using lipofectamine RNAiMAX (Invitrogen). After 48 h, total RNA was extracted and was used as a template for cDNA synthesis. Twenty-five nanograms of the synthesized cDNA was used for RT–PCR amplification with specific primers. PCR products were separated on a 2–3% agarose gel ( Supplementary Figs 6 and 7 ). Immunoblot analysis Cells were lysed in radioimmunoprecipitation assay buffer, and proteins were quantified using a BCA Protein Assay (Pierce). Equal amounts were separated on SDS–polyacrylamide gel electrophoresis gels. Proteins were transferred to nitrocellulose membranes followed by immunoblotting with specific primary antibodies for SF3B1 (1:1,000; #170854; Abcam), Flag (1:1,000, #3165; Sigma), U2AF1 (1:500; #19961; Santa Cruz Biotechnology), U2AF2 (1:500; #53942; Santa Cruz Biotechnology) and β-actin (1:2,000; #5313; Sigma). The membrane was then incubated at room temperature for 1 h with either goat anti-rabbit or goat anti-mouse Odyssey secondary antibodies coupled to a 700 or 800 nm. Immunolabelled proteins were detected using the Odyssey Infrared Imaging System (Li-cor). Quantifications were performed using the ImageJ Software. β-Actin immunoblotting was used to quantify and normalize results. Co-immunoprecipitation HEK293T cells were co-transfected with pcDNA3.11.Myc-U2AF2, kindly given by Edwin Chan [32] , and either pCMV-3tag-1A-SF3B1 WT or pCMV-3tag-1A-SF3B1 K700M . After 48 h, proteins immunoprecipitated by anti-Flag gel affinity (A2220, Sigma) were separated by SDS–polyacrylamide gel electrophoresis and probed in a western blot assay with anti-U2AF2 and anti-U2AF1 antibody ( Supplementary Fig. 8 ). Fragment analysis by capillary electrophoresis Minigene fragments were amplified by RT–PCR using a 5' FAM-forward primer and reverse-specific primers ( Supplementary Table 2 ). One microlitre of RT–PCR product was added to 18.5 μl of deionized formamide and 0.5 μl HD400 marker (Applied Biosystems). The mixture was then denatured 3 min at 95 °C, immediately put on ice, and separated using an ABI 3130xl Genetic Analyzer. The data were analysed using GeneMarker software (SoftGenetics). Accession codes : The RNA-seq data have been deposited in the ArrayExpress repository under the accession code E-MTAB-4097 . How to cite this article : Alsafadi, S. et al . Cancer-associated SF3B1 mutations affect alternative splicing by promoting alternative branchpoint usage. Nat. Commun. 7:10615 doi: 10.1038/ncomms10615 (2016).